A novel gene required for male fertility and functional CATSPER channel formation in spermatozoa Calcium signalling is critical for successful fertilization. In spermatozoa, capacitation, hyperactivation of motility and the acrosome reaction are all mediated by increases in intracellular Ca 2+ . Cat ion channels of sper m proteins (CATSPERS1–4) form an alkalinization-activated Ca 2+ -selective channel required for the hyperactivated motility of spermatozoa and male fertility. Each of the CatSper1–4 genes encodes a subunit of a tetramer surrounding a Ca 2+ -selective pore, in analogy with other six-transmembrane ion channel α subunits. In addition to the pore-forming proteins, the sperm Ca 2+ channel contains auxiliary subunits, CATSPERβ and CATSPERγ. Here, we identify the Tmem146 gene product as a novel subunit, CATSPERδ, required for CATSPER channel function. We find that mice lacking the sperm tail-specific CATSPERδ are infertile and their spermatozoa lack both Ca 2+ current and hyperactivated motility. We show that CATSPERδ is an essential element of the CATSPER channel complex and propose that CATSPERδ is required for proper CATSPER channel assembly and/or transport. Direct recordings of mammalian spermatozoa combined with targeted genetic disruption enabled the precise identification of the sperm ion channel currents that bring calcium into the cell [1] . All mammals and some invertebrate species, contain the genes encoding the alkalinization-activated Ca 2+ -selective ion channels, Cat ion channel of sper m ( CatSpers1–4 ). Genetic deletion of any of the four CatSper genes in mice results in loss of hyperactivated motility and male infertility [2] , [3] , [4] , [5] , [6] , [7] . Biochemical studies show that CATSPERS form a heteromeric complex, likely with each of the CATSPERS1–4 subunits surrounding a central Ca 2+ selective pore, in analogy with other six-transmembrane (6TM) spanning ion channel α subunits [8] . Mutations in CatSper1 and 2 are associated with male infertility in humans [9] , [10] , [11] . In addition to the pore-forming proteins, the sperm Ca 2+ channel contains the auxiliary subunits, CATSPERβ and CATSPERγ [12] , [13] . High amplitude and highly curved movements of the tail characterize hyperactivated motility, which is acquired during capacitation. Hyperactivation serves to generate more force to escape impediments and penetrate barriers such as the zona pellucida [6] , [14] . High pH, cyclic nucleotides, zona pellucida glycoproteins and BSA all can induce CATSPER-dependent Ca 2+ influx [1] , [6] , [15] , [16] . Despite extensive characterization of the functional importance of mutant mice of the CATSPER pore-forming α subunits in male infertility, the difficulty of expressing functional CATSPER channels in heterologous systems, singly or in combination, has limited our understanding of the precise mechanism of CATSPER regulation. Studies suggest that the CATSPER complex includes CATSPERS1–4, CATSPERβ, CATSPERγ and that the complex associates with the chaperone HSPA2 (previously known as HSP70-2) [5] , [12] , [13] . CATSPERβ and CATSPERγ express normally in the testis, but not in spermatozoa of CatSper1-null mice [12] , [13] , suggesting that only a correctly assembled CATSPER channel with all subunits traffic to the flagellar membrane of spermatozoa. Attempts to express functional CATSPER channels in heterologous systems, including Xenopus oocytes with all known six CATSPERS coexpressed with HSPA2, have not been successful. Our working hypothesis is that this failure of heterologous expression is due to the lack of sperm-specific intraflagellar transport machinery and adaptor proteins in these systems. Alternatively, there may be unidentified channel subunits required for proper assembly. To further characterize the CATSPER complex, we performed proteomic analyses with tandem affinity purification followed by mass spectrometry (MS). As a result of these attempts, we identified a novel auxiliary subunit, CATSPERδ (TMEM146), and verified the previously reported CATSPERβ [12] and CATSPERγ [13] auxiliary subunits in the CATSPER complex. CatSperβ , CatSperγ and CatSperδ mRNAs appear in unison 6d before CatSper1 subunit mRNAs in young mice. In mice lacking CatSperδ , CATSPERβ and CATSPERγ form a stable complex, whereas CATSPER1 is substantially reduced, suggesting that CATSPERδ is important for the stability of CATSPER1 and CATSPER complex formation. Most importantly, CatSperδ-null mice spermatozoa lack I CatSper , fail to hyperactivate and are infertile, demonstrating that CATSPERδ is required for proper CATSPER complex formation and ion channel function. Here, we demonstrate that the murine Tmem146 gene encodes CATSPERδ, a critical subunit of the CATSPER ion channel complex. Targeted disruption of CatSperδ abrogated CatSper current, hyperactivated motility and male fertility. We show CATSPERδ association with CATSPER1 is essential for the stability of the CATSPER1 protein before intraflagellar transport and/or incorporation of the CATSPER channel complex into the flagellar membrane. Proteomic identification of CATSPER complex proteins We purified a CATSPER1-containing protein complex from solubilized mouse testes microsomes. To perform purification, we took advantage of the abundance of histidines in the amino terminus of CATSPER1 (51/250 amino acids in the amino terminus) by using metal chelation chromatography and then further enriched the CATSPER1-containing molecular complex by immunoaffinity chromatography with anti-CATSPER1-specific antibody. Proteins of the purified anti-CATSPER1 complex were resolved on SDS–polyacrylamide gel electrophoresis ( Fig. 1a , α-CATSPER1). Numbered protein bands were excised from the gel, digested with trypsin and identified using MS. 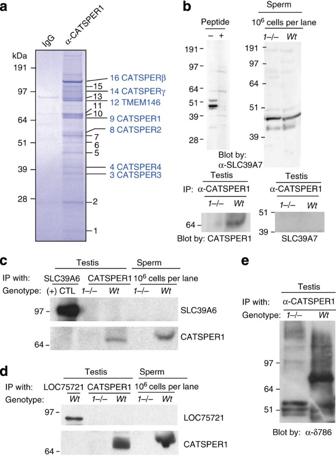Figure 1: Identification of CATSPERδ encoded byTmem146as an auxiliary subunit of native CATSPER channels. (a) Purified CATSPER1 complex (α-CATSPER1) separated by SDS–polyacrylamide gel electrophoresis and stained with Coomassie blue. Rabbit IgG column eluate serves as control (IgG). Numbered protein bands in the purified CATSPER1 complex were subjected to mass spectrometry identification. Confirmed CATSPER1 interactors are listed (blue). The CATSPER channel in the testis is comprised of a macromolecular complex of all four α subunits (CATSPERS1–4), two previously identified auxiliary subunits (CATSPERβ and γ) and a novel auxiliary subunit, TMEM146 (CATSPERδ). (b,c) Two transmembrane proteins that did not express specifically in testes, SLC39A7 (band 5) and SLC39A6 (band 12), were tested for potential interaction with CATSPER1. Anti-SLC39A7 antibody recognized protein in spermatozoa, but its expression was not CATSPER1-dependent. Interaction with CATSPER1 was not found in testis (b). SLC39A6 antibody detected recombinant protein expressed in HEK293T cells ((+) CTL), but no protein was detected in sperm cells or in the CATSPER1 complex (c). (d,e) Two novel testis-specific proteins from band 12 were tested for potential interaction with CATSPER1. LOC75721 was expressed in testis but not in the CATSPER1 immune complex or sperm cells (d). Another protein identified from band12, TMEM146/CATSPERδ co-immunoprecipitates with CATSPER1 (e). Among the identified proteins, confirmed CATSPER1 interactors are listed in Figure 1a . The complete list of proteins that copurified with CATSPER1 is provided in Table 1 . The previously reported CATSPERS1–4 and its auxiliary subunits, CATSPERβ, CATSPERγ and HSPA2 were identified in the purified CATSPER1 molecular complex. Figure 1: Identification of CATSPERδ encoded by Tmem146 as an auxiliary subunit of native CATSPER channels. ( a ) Purified CATSPER1 complex (α-CATSPER1) separated by SDS–polyacrylamide gel electrophoresis and stained with Coomassie blue. Rabbit IgG column eluate serves as control (IgG). Numbered protein bands in the purified CATSPER1 complex were subjected to mass spectrometry identification. Confirmed CATSPER1 interactors are listed (blue). The CATSPER channel in the testis is comprised of a macromolecular complex of all four α subunits (CATSPERS1–4), two previously identified auxiliary subunits (CATSPERβ and γ) and a novel auxiliary subunit, TMEM146 (CATSPERδ). ( b , c ) Two transmembrane proteins that did not express specifically in testes, SLC39A7 (band 5) and SLC39A6 (band 12), were tested for potential interaction with CATSPER1. Anti-SLC39A7 antibody recognized protein in spermatozoa, but its expression was not CATSPER1-dependent. Interaction with CATSPER1 was not found in testis ( b ). SLC39A6 antibody detected recombinant protein expressed in HEK293T cells ((+) CTL), but no protein was detected in sperm cells or in the CATSPER1 complex ( c ). ( d , e ) Two novel testis-specific proteins from band 12 were tested for potential interaction with CATSPER1. LOC75721 was expressed in testis but not in the CATSPER1 immune complex or sperm cells ( d ). Another protein identified from band12, TMEM146/CATSPERδ co-immunoprecipitates with CATSPER1 ( e ). Full size image Table 1 Proteomic analysis of proteins copurified with CATSPER1. Full size table A number of purified molecules were eliminated from consideration as CATSPER complex proteins. Among these were two members of solute carrier family, SLC39A6 and SLC39A7. As these proteins were not testis-specific and did not interact specifically with CATSPER1 ( Fig. 1b,c ), they were likely enriched during purification simply because of the abundance of their histidine residues. Two previously unidentified candidate proteins were detected from band 12; the unannotated hypothetical protein, LOC75721 (NP_898936, accession No. 34147101) and the uncharacterized protein annotated as TMEM146 (accession No. 261245039). Hypothetical protein LOC75721 has no mammalian orthologs and has no transmembrane domains. Despite its expression in the testis, it was not found in the CATSPER1 immune complex, nor was it expressed in spermatozoa ( Fig. 1d ). In contrast, a polyclonal antibody to the very carboxy (C)-terminal region of TMEME146 (RRVKDQNRGKVRVAQKHPET) specifically recognized the ∼ 85 kDa TMEM146 protein in CATSPER1 immunoprecipitates, confirming association of the two proteins ( Fig. 1e ). Analysis of amino acid sequences predicted that TMEM146 has one putative transmembrane domain, but no homology to any other proteins of known function. We refer to the Tmem146 gene product as CATSPERδ. Cloning of CatSperδ Among the many tissues examined, CatSperδ mRNA was detected only in testis ( Fig. 2a ), as previously found for CatSpers1–4 , CatSperβ and CatSperγ [4] , [5] , [6] , [12] , [13] , [17] . The initial mouse Tmem146 cDNA sequences were identified from database searches using novel peptide sequences from MS. These predicted polypeptides (AK077082: 448 amino acids and XM_001052081: 486 amino acids) were much smaller than that predicted from the apparent molecular weight of the band observed in Figure 1e or that predicted for human TMEM146 (798 amino acids, see Supplementary Fig. S1 ). Moreover, the two cDNAs shared a common C-terminus homologous to the C-terminus of human TMEM146. Therefore, 5′-RACE was used to extend the open reading frame (ORF) and reverse transcription–PCR (RT–PCR) was performed to further characterize the two potential splice variants identified. Two products differing by 118 bp were amplified ( Fig. 2b and Supplementary Fig. S1 ). The 118 bp insertion in the 5′-UTR of the small transcript creates a new start site in the ORF. The longer splice variant encodes a protein similar in size to other mammalian Tmem146 orthologues ( Tmem146-l , Supplementary Fig. S1 ). Whole ORFs of the mouse Tmem146 gene were identified by PCR of mouse testis first strand cDNAs ( Fig. 2c ). The PCR product between 2 and 2.5 kbp was cloned and sequenced, yielding Tmem146-l and Tmem146-s . The nucleotide sequences of Tmem146-l (accession no. HQ441159 ) and Tmem146-s (accession no. HQ441160 ) were deposited into GenBank. We conclude that the mouse Tmem146 gene located on mouse chromosome 17 consists of 22 exons and expresses at least two potential splice variants that can encode protein isoforms of 661 (TMEM146-s) and 805 (TMEM146-l) amino acids in length ( Fig. 2d,e ). 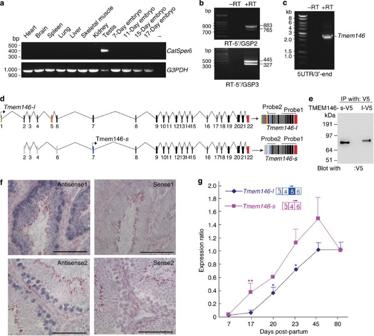Figure 2: Molecular cloning of two alternative splice variants ofCatSperδ. (a) Tissue distribution ofCatSperδmRNA by reverse-transcription PCR.CatSperδ(upper) andGlyceraldehyde 3-Phosphate Dehydrogenase(G3PDH, control; lower) from 12 mouse cDNAs; negative control (lane'–').CatSperδwas detected only in testis. (b,c) Molecular cloning ofCatSperδcDNAs. Two bands differing by 118 bp were amplified by mouse testis first-strand cDNAs by PCR with primers corresponding to the most upstream 5′ sequence identified by 5′-RACE and two different gene-specific primers (GSPs) nested at the 5′-UTR ofTmem146-s. RT, reverse transcriptase (b). Whole open reading frames (ORFs) ofTmem146were amplified from testis cDNA (c). (d) Schematic diagram ofCatSperδsplice variants. Two alternatively spliced mRNA variants are transcribed from theTmem146gene.Tmem146-shas a start site in exon 7 (blue).Tmem146-lcontains a new start site in exon 1 (green) due to a change in the ORF by the additional 118 bp exon 5 (orange). The locations of probes forin situhybridization are illustrated above the transcripts. Probe 1 is complementary to bothTmem146-sandTmem146-l. Probe 2 was amplified fromTmem146-scDNA and corresponds to the splicing region (spanning exon 4 and 6). (e) Heterologous expression of CATSPERδ isoforms. V5-taggedTmem146-sorTmem146-lcDNAs were transfected into HEK293T cells. After immunoprecipitation (IP) with anti-V5, immune complexes were probed with anti-V5. (f) Spatial localization ofTmem146splice variants. Representative fields ofin situhybridization in mouse testis using antisense 1 (upper left) and antisense 2 (lower left). Sense probes served as background controls (right panels). Scale bar, 100 μm. (g) TemporalTmem146-sandTmem146-lmRNA levels (real-time RT–PCR) during testis postnatal development. mRNAs are normalized to TATA-binding protein (TBP) at each time point and expressed as ratios relative to adult (80-day) mouse testis (±s.e.m. compared with each previous time point,*P<0.05,**P<0.005).Tmem146-smRNA was detected at postnatal day 17 (unpaired two-tailedt-test,P=0.0017), whereasTmem146-lappeared at postnatal day 20 (P=0.047 at 20 days,P=0.042 at 23 days), consistent with thein situhybridization experiments. Results are from three independent experiments. Figure 2: Molecular cloning of two alternative splice variants of CatSperδ . ( a ) Tissue distribution of CatSperδ mRNA by reverse-transcription PCR. CatSperδ (upper) and Glyceraldehyde 3-Phosphate Dehydrogenase (G3PDH, control; lower) from 12 mouse cDNAs; negative control ( lane '–'). CatSperδ was detected only in testis. ( b , c ) Molecular cloning of CatSperδ cDNAs. Two bands differing by 118 bp were amplified by mouse testis first-strand cDNAs by PCR with primers corresponding to the most upstream 5′ sequence identified by 5′-RACE and two different gene-specific primers (GSPs) nested at the 5′-UTR of Tmem146-s . RT, reverse transcriptase ( b ). Whole open reading frames (ORFs) of Tmem146 were amplified from testis cDNA ( c ). ( d ) Schematic diagram of CatSperδ splice variants. Two alternatively spliced mRNA variants are transcribed from the Tmem146 gene. Tmem146-s has a start site in exon 7 (blue). Tmem146-l contains a new start site in exon 1 (green) due to a change in the ORF by the additional 118 bp exon 5 (orange). The locations of probes for in situ hybridization are illustrated above the transcripts. Probe 1 is complementary to both Tmem146-s and Tmem146-l . Probe 2 was amplified from Tmem146-s cDNA and corresponds to the splicing region (spanning exon 4 and 6). ( e ) Heterologous expression of CATSPERδ isoforms. V5-tagged Tmem146-s or Tmem146-l cDNAs were transfected into HEK293T cells. After immunoprecipitation (IP) with anti-V5, immune complexes were probed with anti-V5. ( f ) Spatial localization of Tmem146 splice variants. Representative fields of in situ hybridization in mouse testis using antisense 1 (upper left) and antisense 2 (lower left). Sense probes served as background controls ( right panels ). Scale bar, 100 μm. ( g ) Temporal Tmem146-s and Tmem146-l mRNA levels (real-time RT–PCR) during testis postnatal development. mRNAs are normalized to TATA-binding protein (TBP) at each time point and expressed as ratios relative to adult (80-day) mouse testis (±s.e.m. compared with each previous time point, *P <0.05, **P <0.005). Tmem146-s mRNA was detected at postnatal day 17 (unpaired two-tailed t -test, P =0.0017), whereas Tmem146-l appeared at postnatal day 20 ( P =0.047 at 20 days, P =0.042 at 23 days), consistent with the in situ hybridization experiments. Results are from three independent experiments. Full size image Restricted expression of CatSperδ mRNAs in testis To determine the expression pattern of CatSperδ mRNA within testis, we performed in situ hybridization. Two RNA probes were generated by nested PCR amplification of different regions of Tmem146-s cDNA by incorporation of T7 and SP6 RNA polymerase promoters [18] . A single RNA band was observed from each in vitro transcription. Probe 1, complementary to exons 14–22, was used to recognize both Tmem146-s and Tmem146-l transcripts ( Fig. 2d ) and detected CatSperδ in spermatocytes and spermatids in different stages of spermatogenesis ( Fig. 2f ). This expression pattern is similar to that reported for CatSperβ and CatSperγ [12] , [13] . Probe 2 was designed to span the splice junction of exon 4 and 6 of Tmem146-s mRNA, the region unique to the Tmem146-s sequence ( Fig. 2d ). Probe 2 revealed more restricted expression at an early stage of spermatogenesis ( Fig. 2f ), suggesting that Tmem146-s mRNA expression occurs before Tmem146-l . Interstitial cells were not labelled by in situ hybridization by either probe. Using real-time PCR, Tmem146-s mRNA was first detected at postnatal day 17, whereas Tmem146-l appeared at postnatal day 20 of testis development ( Fig. 2g ), consistent with the in situ hybridization experiments. CATSPERδ is a single transmembrane-spanning protein of the sperm tail Mouse CATSPERδ encoded by Tmem146-l is predicted to be 805 amino acids in length with a predicted molecular weight of 91 kDa (pI 6.68; Fig. 3a ). Hydrophilicity plots of mouse and human CATSPERδ suggest that mouse CATSPERδ has one signal peptide, a large extracellular domain of 699 amino acids followed by a transmembrane-spanning domain and ending in an intracellular tail of 60 amino acids ( Fig. 3b ). The predicted transmembrane topology is similar to CATSPERγ. The amino acid sequence of mouse CATSPERδ is not similar to any other protein with known function. CATSPERs1–4, CATSPERβ and CATSPERγ subunits have the same evolutionary pattern; their orthologs are present in the genomes of mammals, as well as sea squirts ( Ciona intestinalis) , and sea urchins ( Strongylocentrotus purpuratus ) [19] . In contrast, CatSperδ orthologues were found only in mammals and a reptile ( Anolis carolinensis , a green lizard), implying that CatSperδ imparts a species-specific function. Like many gamete-specific proteins [19] , CATSPERδ shows signs of rapid evolutionary change as sequence identity between human and mouse CATSPERδ is relatively low (51%; Supplementary Fig. S1 ). 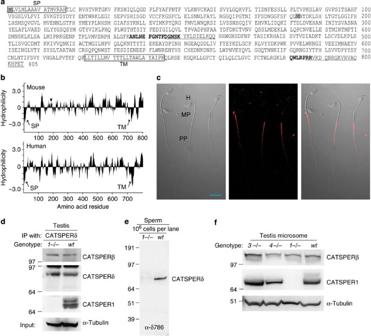Figure 3: Characterization of the CATSPERδ protein. (a) Predicted mouse CATSPERδ protein sequences. Predicted signal peptide (SP) and transmembrane (TM) domain are boxed. The two peptides identified by mass spectrometry are in bold (amino acids 436–450 and 781–787). Two peptide epitopes used to generate antibodies are underlined (amino acids 446–470 and 786–805). The first methionines of two potential TMEM146 isoforms are shadowed in grey. (b) Hydrophilicity plots (window size, 11) of mouse (upper) and human (lower) CATSPERδ. The predicted signal peptide and single transmembrane domain (TM) are marked by arrows. The alternative start site ofTmem146-sis marked by the arrowhead. (c) Immunostaining of mouse sperm by α-CATSPERδ (α-δ446). Left, phase contrast image. The head (H), midpiece (MP) and principal piece (PP) of the sperm are indicated. Middle, immunofluorescence; right, merged signal. Scale bar, 10 μm. (d) Interaction of CATSPER1, CATSPERβ and CATSPERδ inwttestes (wt). CATSPERδ is associated with CATSPERβ regardless of CATSPER1 expression (1−/−). α-Tubulin; input control. (e) Absence of CATSPERδ protein inCatSper1-nullspermatozoa. (f) Expression of CATSPER1 and CATSPERβ in the testis of homozygous nullCatSper1(1−/−),CatSper3(3−/−) andCatSper4(4−/−) and wild-type (wt) mice. Figure 3: Characterization of the CATSPERδ protein. ( a ) Predicted mouse CATSPERδ protein sequences. Predicted signal peptide (SP) and transmembrane (TM) domain are boxed. The two peptides identified by mass spectrometry are in bold (amino acids 436–450 and 781–787). Two peptide epitopes used to generate antibodies are underlined (amino acids 446–470 and 786–805). The first methionines of two potential TMEM146 isoforms are shadowed in grey. ( b ) Hydrophilicity plots (window size, 11) of mouse (upper) and human (lower) CATSPERδ. The predicted signal peptide and single transmembrane domain (TM) are marked by arrows. The alternative start site of Tmem146-s is marked by the arrowhead. ( c ) Immunostaining of mouse sperm by α-CATSPERδ (α-δ446). Left, phase contrast image. The head (H), midpiece (MP) and principal piece (PP) of the sperm are indicated. Middle, immunofluorescence; right, merged signal. Scale bar, 10 μm. ( d ) Interaction of CATSPER1, CATSPERβ and CATSPERδ in wt testes ( wt ). CATSPERδ is associated with CATSPERβ regardless of CATSPER1 expression ( 1 −/− ). α-Tubulin; input control. ( e ) Absence of CATSPERδ protein in CatSper1-null spermatozoa. ( f ) Expression of CATSPER1 and CATSPERβ in the testis of homozygous null CatSper1 ( 1 −/− ), CatSper3 ( 3 −/− ) and CatSper4 ( 4 −/− ) and wild-type ( wt ) mice. Full size image CATSPERδ is strictly localized to the principal piece of spermatozoa ( Fig. 3c ), like all other CATSPER ion channel complex proteins [5] , [6] , [7] , [12] , [13] . CATSPERδ was detected in wild-type ( wt ) and CatSper1-null testis ( Fig. 3d ), but not in mature CatSper1-null spermatozoa ( Fig. 3e ). This result is concordant with CATSPERβ and CATSPERγ expression in mice lacking CatSper1 [12] , [13] (see also Fig. 3d,f ). Thus, the expression of auxiliary subunits of CATSPER channel in sperm cells depends on the presence of CATSPER1 and presumably other pore-forming α subunits, suggesting that complete and proper assembly of CATSPER channel complex is a prerequisite to intraflagellar trafficking, insertion of the complex into the flagellar membrane, or both. Targeted disruption of CatSperδ As reconstitution of functional CATSPER channels has not succeeded in any heterologous system, genetic manipulation remains the primary tool to study the function of CATSPER subunits. Interestingly, mouse CatSperβ and CatSperγ genes were duplicated at some point in evolution. CatSperβ and its partial duplicate are separated by ∼ 37 kbp apart on chromosome 12, whereas copies of CatSperγ are separated by 480 kbp on chromosome 7. These duplications complicate genetic disruption of CatSperβ and CatSperγ . In contrast, only a single copy of CatSperδ is found in the mouse genome. Thus, we generated a CatSperδ-null mouse line lacking CATSPERδ using the recombineering technique [20] . Following homologous recombination, exon 9 was excised by Cre -recombinase in embryonic stem (ES) cells ( Fig. 4a ). Deletion of exon 9 resulted in a frame-shift and generated multiple downstream stop codons, thereby inactivating both Tmem146-s and Tmem146-l transcripts ( Fig. 4a and Supplementary Fig. S1 ). PCR screening of flanking regions of the targeting construct revealed clones with successful homologous recombination ( Fig. 4b ). Deletion of exon 9 was confirmed in the smaller PCR product of the genomic sequence in the Cre -catalysed ES clone ( Fig. 4c , 97-Cre ). Absence of exon 9 in the CatSperδ transcript of homozygous null mice was confirmed by RT–PCR of testis mRNA ( Fig. 4d ). No CATSPERδ was detected in CatSperδ-null spermatozoa as determined by immunocytochemistry ( Fig. 4e ) and immunoblotting ( Fig. 4f ). 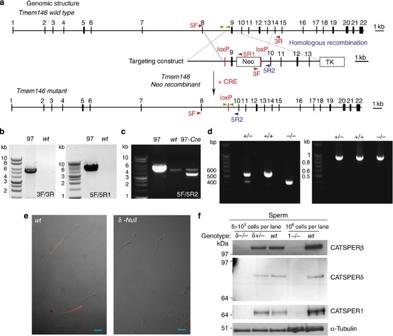Figure 4: Targeted disruption ofTmem146gene inactivatesCatSperδ. (a) Whole genomic structure of mouseTmem146gene, targeting construct and predicted mutant allele generated by homologous recombination andCreexcision; Filled boxes, exons; thin lines, introns. Neomycin (Neo) and thymidine kinase (TK) selection cassettes are shown. The locations of primers used for genotyping are shown with arrowheads. Primers located outside targeting region, 5F and 3R; inside targeting region, 5R2; withinNeo, 5R1 and 3F. (b,c) PCR genotyping of genomic DNA.Tmem146 Neomutant ES clone (97) is identified by the presence of PCR products at both the 3′- (3F/3R) and 5′- (5F/5R2) of the expected locus (b). Excision of genomic sequence flanked by twoloxPsites by PCR with 5F/5R2 (c). (d) RT–PCR ofCatSperδwith testis mRNA fromCatSperδ−nullmice showing the expected products. Combination of two primers with one spanning exon 7/8 and the other in exon 12 demonstrates absence of exon 9 in theCatSperδtranscript (left). RT–PCR ofGAPDHis the control (right),CatSperδ-null(−/−),CatSperδ-heterozygotes(+/−) and wild type (+/+). (e) Immunostaining of mouse epididymal sperm with anti-CATSPERδ antibody (α-δ446). CATSPERδ specifically labels only the principal piece of the tail ofwtspermatozoa (left) and is not observed in theCatSperδ-nullsperm cells (right). Scale bar, 10 μm. (f) Absence of CATSPER1, β and δ proteins in spermatozoa ofCatSperδhomozygous null mice. Figure 4: Targeted disruption of Tmem146 gene inactivates CatSperδ . ( a ) Whole genomic structure of mouse Tmem146 gene, targeting construct and predicted mutant allele generated by homologous recombination and Cre excision; Filled boxes, exons; thin lines, introns. Neomycin (Neo) and thymidine kinase (TK) selection cassettes are shown. The locations of primers used for genotyping are shown with arrowheads. Primers located outside targeting region, 5F and 3R; inside targeting region, 5R2; within Neo , 5R1 and 3F. ( b , c ) PCR genotyping of genomic DNA. Tmem146 Neo mutant ES clone (97) is identified by the presence of PCR products at both the 3′- (3F/3R) and 5′- (5F/5R2) of the expected locus ( b ). Excision of genomic sequence flanked by two loxP sites by PCR with 5F/5R2 ( c ). ( d ) RT–PCR of CatSperδ with testis mRNA from CatSperδ−null mice showing the expected products. Combination of two primers with one spanning exon 7/8 and the other in exon 12 demonstrates absence of exon 9 in the CatSperδ transcript (left). RT–PCR of GAPDH is the control (right), CatSperδ-null (−/−), CatSperδ-heterozygotes (+/−) and wild type (+/+). ( e ) Immunostaining of mouse epididymal sperm with anti-CATSPERδ antibody (α-δ446). CATSPERδ specifically labels only the principal piece of the tail of wt spermatozoa (left) and is not observed in the CatSperδ-null sperm cells (right). Scale bar, 10 μm. ( f ) Absence of CATSPER1, β and δ proteins in spermatozoa of CatSperδ homozygous null mice. Full size image CatSperδ is required for male fertility CatSperδ-null mutant mice are indistinguishable from their wt or heterozygous ( het ) littermates in appearance, gross behaviour and survival. In addition, no morphological differences were observed by histological examination of testis and epididymis ( Fig. 5a ). CatSperδ-null female mice exhibited normal mating behaviour and gave birth to litters comparable to those of wt females when mated with wt or het males. However, when CatSperδ-null male mice were mated with wt or het females (four pairs for >3 months), no litters was produced, indicating that CatSperδ-null male mice are completely infertile. In contrast, 18 litters were produced as offspring of 5 pairs of heterozygous males and females, yielding 128 pups (31 wt , 67 het and 30 null ) in a Mendelian ratio with an average of 7.1 pups per litter during the same period ( Fig. 5b ), and similar to 7.8 pups per litter for wt mice [5] . The sperm count from CatSperδ homozygous null mice was slightly lower than that of paired littermate heterozygous mice at 2–3 months of age, but was not significantly different at 7–8 months of age ( Fig. 5c ). Tmem146/CatSperδ is reportedly reduced in tetrazoospermic patients (GDS2697/237020_at/Tmem146 in Gene Expression Omnibus (GEO) profiles) [21] , but more studies are warranted to examine the roles of the two isoforms during early spermatogenesis. 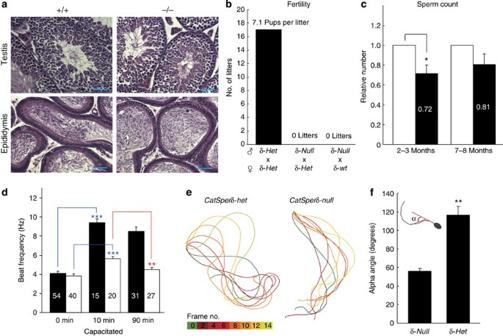Figure 5:CatSperδ-nullmale mice are infertile and their sperm fail to hyperactivate. (a) Hematoxylin and eosin staining of the testes (top) and epididymis (bottom) ofwt(left) andCatSperδ-null(right) mice. Testis morphology is normal. Scale bar, 50 μm. (b)CatSperδ-nullmales are infertile. (c) Epididymal sperm count (mean±s.e.m.) from littermates at ages of 2–3 or 7–8 months of age (six pairs each).Het(open) versusnull(filled): *P<0.05, paired two-tailedt-test. (d) Flagellar beat frequency ofCatSperδ-het(open) andnullsperm (filled). Basal beat frequency immediately after isolation (time 0), beat frequencies of activated (10 min) and hyperactivated (90 min) sperm cells incubated in capacitating media;n=15–54 tethered sperm cells in four independent experiments (unpaired two-tailedt-test, ***P<0.001, **P<0.005). (e) Aligned flagellar waveform traces. Sperm cells were examined 90 min after incubation in capacitating conditions to induce hyperactivation. Representative traces of single spermatozoa ofCatSperδ-hetandCatSperδ-nullare shown.CatSperδ-hetfull beat cycle lasted for∼230 ms, during whichCatSperδ-nullsperm completed two beat cycles. (f) Measurement of bending angle. Capacitatedhetspermatozoa exhibit larger ranges of motion thanCatSperδ-nullspermatozoa as indicated by the maximum bending angle (inset, α; unpaired two-tailedt-test, **P<0.005).n=6. Figure 5: CatSperδ-null male mice are infertile and their sperm fail to hyperactivate. ( a ) Hematoxylin and eosin staining of the testes (top) and epididymis (bottom) of wt ( l eft) and CatSperδ-null ( r ight) mice. Testis morphology is normal. Scale bar, 50 μm. ( b ) CatSperδ-null males are infertile. ( c ) Epididymal sperm count (mean±s.e.m.) from littermates at ages of 2–3 or 7–8 months of age (six pairs each). Het (open) versus null (filled): * P <0.05, paired two-tailed t -test. ( d ) Flagellar beat frequency of CatSperδ - het (open) and null sperm (filled). Basal beat frequency immediately after isolation (time 0), beat frequencies of activated (10 min) and hyperactivated (90 min) sperm cells incubated in capacitating media; n =15–54 tethered sperm cells in four independent experiments (unpaired two-tailed t -test, *** P <0.001, ** P <0.005). ( e ) Aligned flagellar waveform traces. Sperm cells were examined 90 min after incubation in capacitating conditions to induce hyperactivation. Representative traces of single spermatozoa of CatSperδ - het and CatSperδ-null are shown. CatSperδ - het full beat cycle lasted for ∼ 230 ms, during which CatSperδ-null sperm completed two beat cycles. ( f ) Measurement of bending angle. Capacitated het spermatozoa exhibit larger ranges of motion than CatSperδ-null spermatozoa as indicated by the maximum bending angle (inset, α; unpaired two-tailed t -test, ** P <0.005). n =6. Full size image CatSperδ-null spermatozoa fail to hyperactivate and lack I CatSper Bicarbonate increases mammalian spermatozoa motility by stimulating soluble adenylyl cyclase (ADCY10) [22] , [23] . We tested bicarbonate-evoked activation of motility in CatSperδ-null sperm and found that activated motility was preserved in both CatSperδ-null (9.5±0.4 Hz) and CatSperδ-het (5.7±0.2 Hz) mouse spermatozoa compared with sperm cells under non-capacitating conditions ( Fig. 5d ; time 0 versus 10 min, P =10 −11 for CatSperδ-null ; P =10 −5 for CatSperδ-het sperm, ***; compare Supplementary Movies 1 , 2 , 3 and 4 ). This result is consistent with previous reports showing that CATSPER1 and CATSPER2 are not required for the initial activation of flagellar beating [2] , [3] induced by cAMP after bicarbonate activation of soluble adenylyl cyclase (ADCY10). In contrast, CatSperδ-null sperm fail to develop hyperactivated motility as was also observed in CatSpers1–4 mutant sperm cells (compare Supplementary Movies 5 and 6 ). After 90 min under capacitating conditions, beat frequency significantly decreased in CatSperδ - het spermatozoa (4.6±0.2 Hz) when compared with that of activated sperm (5.7±0.2 Hz; Fig. 5d , 10 versus 90 min, ** P =0.0012). Flagellar amplitudes of CatSperδ-het spermatozoa (and wt , see ref. 3 ) were substantially larger than that of capacitated CatSperδ-null spermatozoa ( Fig. 5e ). In contrast, capacitating conditions did not substantially change the flagellar amplitude of CatSperδ-null spermatozoa (compare Supplementary Movies 3 , 4 , 5 and 6 ). Aligned flagella waveform traces of representative sperm reveal the lower frequency of movement in het spermatozoa (one averaged full beat cycle=225 ms compared with 175 ms in activated sperm cells). In comparison, CatSperδ-null sperm complete one cycle in 108 ms under the same capacitating conditions ( Fig. 5e , Supplementary Fig. S2 ). These changes are consistent with previous reports in CatSper1-null mice [3] . Another well-established feature of hyperactivated spermatozoa is an increase in the angle between head/midpiece and the principal piece known as the bend angle [2] , [5] . In CatSperδ-null mice, the maximum bend angle (α) of the principal bend in the midpiece was 56±3° relative to 0° (straight), significantly smaller than the 117±10° bend angle recorded in het spermatozoa under capacitating conditions ( Fig. 5f , unpaired two-tailed t -test, P =0.0018). I CatSper is a sperm-specific, Ca 2+ -selective, pH-sensitive ion current mediated by CATSPER proteins [1] . I CatSper is small and difficult to record in normal 2 mM Ca 2+ bath solution. As is typical for Ca 2+ -selective channels, this is remedied by recording in divalent-free solution where I CatSper is carried by Na + ions [1] . In CatSperδ-het spermatozoa, I CatSper mediates a large Na + inward current (−950±190 pA at −100 mV; Fig. 6a ), indistinguishable from previously recorded wt spermatozoa [1] . In sperm from CatSperδ-null mice, monovalent CATSPER current was not detected (<−9±8 pA at −100 mV; Fig. 6b ), consistent with the absence of current in mice lacking CatSpers1, 2, 3 or 4 (refs 1 , 5 ). In addition, expression of CatSperδ with CatSper1, 2, 3, 4 , β and γ , as well as Hspa2 , failed to yield detectable ion currents in Xenopus oocytes, suggesting that the CATSPER complex is still incomplete, or that specific flagellar proteins are required for proper membrane insertion of a CATSPER complex. 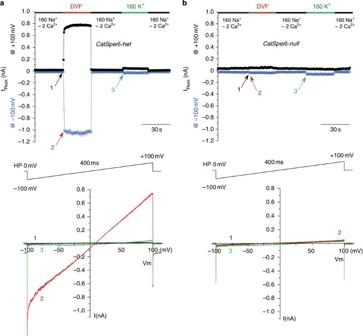Figure 6:CatSperδ-nullmice lack CatSper current. (a)CatSperδ-hetand (b) CatSperδ-null ICatSper. The upper traces show representative time courses ofICatSpermeasured in control solutions (1), nominally divalent-free (DVF) solutions (2), and high-K+solutions (3) at −100 mV (blue circles) and +100 mV (black circles). Bottom panels show the current–voltage relations of monovalentICatSperin response to voltage ramps at the time points indicated.ICatSperis absent inCatSperδ-nullsperm cells. A small inwardIKSperwas seen in both phenotypes when the bath solution was switched to 160 mM K-MeSO3.CatSperδ-hetcurrents are indistinguishable from previously publishedwtcurrents1. Figure 6: CatSperδ-null mice lack CatSper current. ( a ) CatSperδ-het and ( b ) CatSper δ-null I CatSper . The upper traces show representative time courses of I CatSper measured in control solutions (1), nominally divalent-free (DVF) solutions (2), and high-K + solutions (3) at −100 mV (blue circles) and +100 mV (black circles). Bottom panels show the current–voltage relations of monovalent I CatSper in response to voltage ramps at the time points indicated. I CatSper is absent in CatSperδ-null sperm cells. A small inward I KSper was seen in both phenotypes when the bath solution was switched to 160 mM K-MeSO 3 . CatSperδ-het currents are indistinguishable from previously published wt currents [1] . Full size image I KSper is a pH-sensitive K + current in sperm [24] mediated by the mSLO3 (refs 25 , 26 ) and is responsible for hyperpolarization of spermatozoa during capacitation [26] . By hyperpolarizing the spermatozoan membrane potential to −50 mV (refs 8 , 26 ), it increases the driving force for Ca 2+ entry via the CATSPER channel. In CatSperδ-null spermatozoa, I KSper did not differ substantially from heterozygous spermatozoa ( Fig. 6 ). Inactivation of CatSperδ decreases the stability of CATSPER1 CATSPERS3, 4, CATSPERβ and CATSPERγ are expressed in testis, despite their absence in the principal piece of sperm cells in CatSper1-null mice [12] , [13] . In testis, they are present in the endoplasmic reticulum (ER) and the Golgi apparatus, as is typical for proteins during assembly. Similarly, CATSPERδ levels are indistinguishable from wt in the testes of mice lacking CatSper1 . However, CATSPERδ does associate with CATSPERβ in the testis of these mutant mice ( Fig. 3d ). We next examined the expression and association of other CATSPERS in the testis and spermatozoa of CatSperδ-null mice. Strikingly, ablation of CatSperδ dramatically reduced CATSPER1 levels in the testis ( Fig. 7a input). Real-time qRT–PCR results indicate that CatSper1 , CatSperβ and CatSperγ mRNA expression in testes were not substantially different in CatSperδ-null compared with CatSperδ-het mice ( Supplementary Fig. S3 ), suggesting that transcriptional regulation is not responsible for the CATSPER1 reduction observed in CatSperδ-null mice and that CATSPER1 is subject to degradation if not assembled properly with CATSPERδ. Collectively, these data indicate that progression of the CATSPER complex from the Golgi/ER to the flagellar membrane requires proper assembly of the complex. 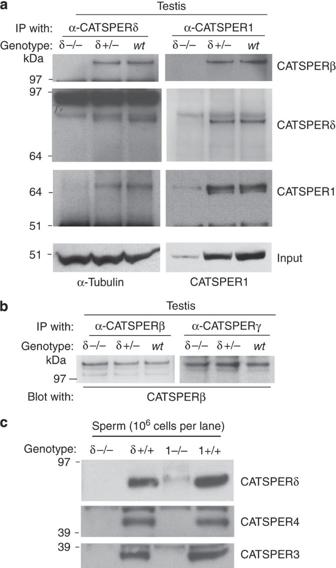Figure 7: Inactivation ofCatSperδdecreases the stability of CATSPER1 during spermatogenesis. (a) Reduction of CATSPER1 protein byCatSperδdeletion. Proteins solubilized from testis are immunoprecipitated (IP) with specific anti-CATSPERδ antibodies (α-δ786, IP, left) or anti-CATSPER1 (IP, right). CATSPERδ was pulled down fromCatSperδ-het(δ+/−) andwt(+/+) testes but not from homozygous mutant testes (δ−/−, IP, left, middle). CATSPERβ and CATSPER1 proteins are found in the same protein complex fromCatSperδ-hetandwttestes (IP, left, top and bottom). Reciprocally, anti-CATSPER1 antibodies also co-immunoprecipitated CATSPERβ and CATSPERδ (IP, right, top and middle) fromCatSperδ-hetandwttestes. The amount of CATSPER1 was greatly reduced in theCatSperδhomozygous mutants (input, right), whereas input control (α-tubulin) was unchanged (input, left). A small amount of CATSPER1 was recovered by anti-CATSPER1 immunoprecipitation from homozygous mutant testes (IP, right, bottom left lane). (b) InCatSperδhomozygous null mice, CATSPERβ was associated with CATSPERγ. (c) Absence of expression of CATSPER3 and CATSPER4 subunits in the sperm cells ofCatSperδhomozygous null mice. Figure 7: Inactivation of CatSperδ decreases the stability of CATSPER1 during spermatogenesis. ( a ) Reduction of CATSPER1 protein by CatSperδ deletion. Proteins solubilized from testis are immunoprecipitated (IP) with specific anti-CATSPERδ antibodies (α-δ786, IP, left) or anti-CATSPER1 (IP, right). CATSPERδ was pulled down from CatSperδ - het ( δ +/− ) and wt (+/+) testes but not from homozygous mutant testes ( δ −/− , IP, left, middle). CATSPERβ and CATSPER1 proteins are found in the same protein complex from CatSperδ-het and wt testes (IP, left, top and bottom). Reciprocally, anti-CATSPER1 antibodies also co-immunoprecipitated CATSPERβ and CATSPERδ (IP, right, top and middle) from CatSperδ - het and wt testes. The amount of CATSPER1 was greatly reduced in the CatSperδ homozygous mutants (input, right), whereas input control (α-tubulin) was unchanged (input, left). A small amount of CATSPER1 was recovered by anti-CATSPER1 immunoprecipitation from homozygous mutant testes (IP, right, bottom left lane). ( b ) In CatSperδ homozygous null mice, CATSPERβ was associated with CATSPERγ. ( c ) Absence of expression of CATSPER3 and CATSPER4 subunits in the sperm cells of CatSperδ homozygous null mice. Full size image mRNA expression of CatSpers1–4 is reportedly developmentally regulated during mouse sexual maturation. CatSper2 mRNA is first detected at postnatal day 18, and the mRNAs of CatSper3 , 4 and 1 follow at postnatal day 21, 21 and 21–25, respectively [29] , [30] . To obtain more insight into the potential roles of CATSPERδ in the assembly, stability or transport of the CATSPER complex, temporal mRNA expression of the β , γ and δ CatSper auxiliary subunits was compared with CatSper1 expression by real-time PCR, during postnatal testis development. mRNA of auxiliary subunits appeared around postnatal day 17, earlier than the initiation of CatSper1 mRNA expression (postnatal day 23, consistent with refs 28 , 29 ; Supplementary Fig. S3 ). These data suggest that CATSPERδ, CATSPERβ and CATSPERγ are likely to be synthesized before and during CATSPER1 expression. The dramatic reduction of CATSPER1 ( Fig. 7a ), the preservation of interaction between other auxiliary subunits in testes of CatSperδ-null mice ( Fig. 7b ), and the absence of all CATSPER proteins in spermatozoa of CatSperδ-null mice ( Figs 4f and 7c ) suggests that CATSPERδ assembly with CATSPER1 is required to prevent CATSPER1 degradation. CATSPERδ may have additional functions in transport and/or membrane insertion of the CATSPER channel complex. CATSPER channels are unique, sperm-specific, Ca 2+ -selective ion channels. As we have shown in previous papers and in the present work, the CATSPER channel is much more complex in its protein composition than all other ion channels to date. First, four independent genes encode each α subunit of the tetrameric Ca 2+ -selective pore, compared with the one α subunit gene encoding the 4×6TM repeat structure of Ca V channels, or the one gene that encodes the tetrameric Ca 2+ -selective channels such as Orai1, TRPV5 or TRPV6. The common theme among all these channels is that the α subunits position the pore lining residues into the centre of the protein, shielding the transfer of charge across the lipid bilayers. Each CATSPERα subunit contains a pair of negatively charged aspartic acid residues that, by inference from work on other Ca 2+ channels, come together to bind Ca 2+ within the pore and confer its Ca 2+ ion selectivity. A second unusual feature of CATSPER channels is that each voltage-sensing domain (S1–S4) differs from the others. In other voltage-sensing channels, the S1–S4 domain contains positively charged (usually arginine) amino acids every third residue in the fourth transmembrane spanning segment (S4). In the CATSPER complex, CATSPER1 generally follows this convention, whereas CATSPERS4, 2 and 3 have increasingly fewer charged residues. The end result is that CATSPER is only weakly voltage sensitive. Perhaps at an early stage of evolution, this voltage-gating property was important, but has been progressively lost. A third unusual feature is CATSPER1's histidine-rich amino terminus. As heterologous expression of the CATSPER complex is not currently possible to conduct mutagenesis studies, we can only surmise that these histidines may be important for CATSPER channel proton sensitivity or Zn 2+ binding. Like CATSPER, Ca V channels have auxiliary subunits, defined as protein subunits that do not directly participate in pore formation. Ca v 1 and Ca V 2 α1 subunit commonly associate with proteins named α2δ and β, but these have no homology to the CATSPER β, γ and δ subunits. The topology of Ca v α2δ is similar to CATSPERs γ and δ in that all three have a single transmembrane-spanning domain and a large extracellular amino-terminal loop. Ca v channel auxiliary subunits are not required for expression, but rather seem to modulate expression levels and channel kinetics [8] , [30] . In contrast, as we have shown here, CATSPERδ is required for CATSPER channel α subunit expression and function. In spermatozoa, the constraints on channel trafficking are more stringent than for other ion channels in non-sperm cells. For the CATSPER complex, seven distinct gene products must be assembled and targeted specifically to the principal piece of the sperm tail. The tail, being a flagellar/ciliary structure, employs an intraflagellar transport system for protein targeting [31] . Thus, one or more of the CATSPER auxiliary subunits may be important for adapting to flagellar transport motors or the complex's insertion into the membrane. Another possibility is that one or more of the auxiliary subunits are important for assembly in the ER or the Golgi apparatus. Although mRNA levels do not accurately report protein levels, all CatSper auxiliary subunit mRNAs appear well before CatSper α subunit mRNAs during postnatal development. In addition, none of the CatSper1, 3 or 4 null mutants affected expression levels of auxiliary subunits ( Fig. 3f ). Thus, one possibility is that the auxiliary subunits must appear before CATSPERα subunits to enable their proper assembly. In support of this notion, CatSperδ ablation resulted in much reduced detected CATSPER1-α subunit, suggesting that one function of the auxiliary subunits may be to prevent CATSPERS 1, 3, or 4 from proteosomal degradation before or during transport. As an example, the voltage-sensing domain of CATSPER1 may require a chaperone during assembly as proposed for ancillary subunits of Kv4 channels [32] . The fact that all the CATSPER auxiliary subunits have large extracellular domains raises the question of whether they bind factors that might initiate or alter CATSPER channel gating. It will be important to understand the structure of these domains and determine whether they bind potential gating agents, such as reproductive hormones (for example, progesterone), chemoattractants or surface recognition molecules. Our study identifies CATSPERδ, encoded by the Tmem146 gene, as being required for male fertility via its crucial role in the CATSPER channel complex. The phenotypes for mice in which any of the CatSper1–4 or CatSperδ genes are ablated are practically identical, with each displaying complete loss of I CatSper and consequent failure of hyperactivated motility, gradual loss of progressive motility over time and complete male infertility. One minor difference seems to be a slight decrease in CatSperδ-null sperm counts in young animals, but a role for CatSperδ isoforms in spermatogenesis will require much more detailed study. As for CatSper1 and 2 (refs 9 , 10 , 11 ), it is likely that human male infertility genes will be found for mutant CatSpers 3, 4, CatSperδ and perhaps CatSperβ and CatSperγ. With seven subunits of the CATSPER channel identified and a more thorough understanding of CATSPER trafficking in the future, it may be possible to express a functional channel in heterologous systems to screen compound libraries for contraceptive agents. CATSPER channel complex purification and peptide identification The CATSPER channel complex was purified from mouse testes by affinity chromatography at 4 °C and monitored by CATSPER1 western blotting. A total of 25 frozen mouse testicles (Pel-Freeze Biologicals) were homogenized and microsomes were isolated by step centrifugation in 0.32 M sucrose buffer with protease inhibitor cocktail (PIC, no EDTA; Complete, Roche; yield ∼ 850 mg). Microsomal proteins were solubilized in Tris-buffered saline (TBS)-1% Triton X-100 with PIC and cleared by centrifugation at 100,000 g (yield ∼ 400 mg). Native CATSPER1 bound to cobalt resin (Talon, Clontech) were eluted from an imidazole gradient. Fractions containing CATSPER1 ( ∼ 1 mg protein) were pooled and bound to immobilized anti-CATSPER1 resin (Protein A Sepharose, Amersham). Bound CATSPER1 complex was washed in high-stringency conditions (RIPA+0.2 M imidazole) and eluted in 0.1 M glycine-0.4% CHAPS, pH 2.5. CATSPER1-copurified proteins were separated by 4–12% gradient SDS gel electrophoresis (Invitrogen) and visualized by Coomassie staining. Proteins purified from identical preparations with immobilized preimmune immunoglobulins were considered to be nonspecific. Specific, copurified protein bands were excised and in-gel digested with trypsin. Dried peptides were dissolved in matrix, subjected to matrix-assisted laser desorption/ionization–time of flight MS and MS/MS analyses using a 4,700 Proteomics analyzer and GPS software (Applied Biosystems). A combination of peptide mass fingerprinting and the MS/MS analysis was performed using the Mascot search engine (Matrix Science). Collision-induced dissociation spectra were submitted for protein identification with a precursor precision tolerance of 1 Da and MS/MS fragment tolerance of 0.5 Da. Multiple tissue RT–PCR PCR was performed according to standard protocols using a commercial multiple panel cDNA template (MTC, Clontech). PCR primers amplified Tmem146 from exons 16 to 19 (forward: 5′-TCAACTTCACTGCCAGCATC-3′, reverse: 5′-TCCCATTCTTCCACAGTTCC-3′) using mouse G3PDH as control. Molecular cloning The complete coding sequence of Tmem146 was assembled by 5′ RACE amplification (Marathon Ready Mouse Testis cDNA, Clontech) using cDNA fragment-specific antisense (GSP2: 5′-GATGTTGATGTTGGC-3′ and GSP3: 5′-GGAGCCTTTGAAACAACAAACGTCACCA-3′) and an AP primer. Two splice variants were detected by RT–PCR with the RACE identified 5′-sequence as forward (RT-5′-CAAGATGCTGGTGTTGATGC-3′) and two reverse primers ( Fig. 2b , upper with GSP3 and lower with GSP2). Full-length Tmem146 cDNAs were obtained by RT–PCR with primers to the RT-5′ and 3′-end (5′-CTATGTCTCTGGATGTTTCTGGGCAACTCG-3′). Sequencing the TOPO-cloned PCR products into pCR4-TA (Invitrogen) confirmed the assembled Tmem146 cDNAs. In situ hybridization Paraffin sections (10-μm thick) of 4% paraformaldehyde-fixed mouse testes were probed with digoxigenin-labeled antisense RNA probes. Probe 1 corresponds to 1,078 bp covering exons 14–22 (forward: 5′-GGCAACTCTAAGTACAAACT-3′ and reverse: 5′-ATGTCTCTGGATGTTTCTGGG-3′) and probe 2 corresponds to 448 bp of exons 4/6–10 (excluding exon 5; forward: 5′-CAAGTCATTGGCGGTATATCAG-3′ and reverse: 5′-GCACGTGTTCAACAATCTGG-3′). Antisense probe 2 is completely complementary to the Tmem146-s and forms an antisense-target RNA duplex for detection of the small transcript. Probe 2 is either partially complementary to Tmem146-l , with 13 bp tandem mismatches at its 3′ end, or requires an 118 bp region of bulged nucleotides in Tmem146-l mRNA to form the 3′ duplex. In either case, hybridization of probe 2 with Tmem146-l is thermodynamically less favourable than the hybridization with Tmem146-s (ref. 33 ) and is most likely to report mRNA expression of Tmem146-s . Real-time qRT–PCR analysis for CatSpers expression Real-time PCR was carried out with first strand cDNAs from 2 μg total testis RNA using the SYBR Green (RT2 Real-Time SYBR Green/ROX PCR, SABiosciences; Eppendorf Realplex). Quantitative analysis by the ΔΔ C t method [34] employed TATA box binding protein as amplification controls. Three independent sets of experiments were performed to calculate fold changes ( 2 - Δ Δ C t ) of CatSpers mRNA. The primers used for qRT–PCR were: CatSper1 (forward1: 5′-CTGCCTCTTCCTCTTCTCTG-3′, reverse1: 5′-TGTCTATGTAGATGAGGGACCA-3′ and forward2: 5′-GCAAATGATATTGTCACTGACC-3′, reverse2: 5′-CATGAAGTACCATTCACCTCG-3′), CatSperβ (forward: 5′-CCTTATTGACCAAGAAACAGAC-3′, reverse: 5′-TGAAACCCATATTTGACTGCC-3′), CatSperγ (forward1: 5′-TGAGCAATAGAGGTGTAGAC-3′, reverse1: 5′-CAGGATGTAGAAGACAACCAG-3′ and forward2: 5′-GATCCGTCAGAGAACTATTTGAG-3′, reverse2: 5′-GGAGTCCACCATCAAATACATGG-3′), CatSperδ (forward1: 5′-GAAGCATACGATCCTATCAACC-3′, reverse1: 5′-CCATTCTTCCACAGTTCCAC-3′ and forward2: 5′-GTCGAGTATCAGGTCTTAGG-3′, reverse2: 5′-GTTGCAGTAGCTGTAGTATGG-3′) and TATA box binding protein (forward: 5′-GCTGACCCACCAGCAGTTCAGTA-3′, reverse: 5′-AAGGAGAACAATTCTGGGTTTG-3′). For specific detection of Tmem146 splice variants, Tmem146-l (forward: 5′-GCTGACATTTCTGTGTATCTAGG-3′, reverse: 5′-CTGATATACCTTCCAATTTACGCC-3′), Tmem146-s (forward: 5′-GCTGACATTTCTGTGTATCTAGG-3′, reverse: 5′-CTGATATACCGCCAATGACTTGG-3′). Antibodies Anti-CATSPER1, 3 and 4 antibodies were described [5] , [6] . Peptides corresponding to amino acids 446–459 (α-δ446: DGNSKYKLDIELKQ) and 786–805 (α-δ786: RRVKDQNRGKVRVAQKHPET) of CATSPERδ, 884−899 (TDNFYHADPSKPIPRN) of CATSPERβ and 53−73 (KFEKVGLHLSKDRFQDHEPID) of CATSPERγ, 21–39 (α-LOC75721: DDHQLSESLSEDYDLPDYD) of hypothetical protein LOC75721 (NP_898936), 74–90 (α-SLC39A6: EGFRKLLQNIGIDKIKR) of zinc transporter ZIP6 precursor (SLC39A6), and 29–42 (α-SLC39A7: EGHGDLHKDVEEDF) of zinc transporter SLC39A7 were synthesized and conjugated to KLH carrier protein to produce antiserum (Open Biosystems). The antisera were affinity purified on the immobilized resin of the corresponding peptide (Amino Link plus, Pierce). Anti-V5 and anti-α tubulin antibodies are from Invitrogen and Cell Signaling Technologies, respectively. Immunocytochemistry Sperm cells from the cauda epididymis attached to glass coverslips were fixed in 4% paraformaldehyde in PBS, permeabilized with 0.2% TrixonX-100 for 5 min, washed in PBS and blocked with 10% goat serum for 1 h. Samples were stained overnight with primary antibody against CATSPERδ (a-δ446, 10 μg ml −1 ) in 10% goat serum, 4 °C. After PBS wash, goat-anti-rabbit Alexa568 conjugate (Molecular Probes) served as secondary antibody. Images were acquired by confocal microscopy (Olympus Fluoview 1000). Tmem146 targeting construct and analysis of ES cell clones A mouse Tmem146 gene fragment was isolated from a BAC clone and the targeting construct created by recombineering [20] . Materials for homologous recombination were provided by the NCI-Frederick Institute ( http://recombineering.ncifcrf.gov/ ). The targeting construct was linearized and electroporated into ES cells derived from 129/SvJ1 mice for homologous recombination. G418-resistant colonies were selected and clones carrying mutated Tmem146 genomic sequences at the proper locus (5F: 5′-GAGGTTCAATTTCCAGCAGTC-3′, 5R1: 5′-GACGTGCTACTTCCATTTGTC-3′, 3F: 5′-TACCCGTGATATTGCTGAAGAG-3′, 3R: 5′-GGAGGGAGATAGACAAGACAC-3′) were identified. The ES cell clone harbouring the targeting construct (clone 97) were transfected with pOG231, a plasmid for transient Cre expression, to excise the neomycin cassette and create the conditional null allele. Subsequent subclones (clones 97- Cre ) with the appropriate recombination of loxP sites were genotyped (5F: 5′-GAGGTTCAATTTCCAGCAGTC-3′, 5R2: 5′-GTGATGACCCATAAATGTTGCC-3′). Generation of CatSperδ -deficient mice and genotyping of mutant mice Three mutant ES cell clones (97- Cre ) were injected into C57BL/6 blastocysts and transplanted into the uterus of pseudopregnant foster mothers. Chimeric animals were bred with C57BL/6 to obtain heterozygous offspring. Initially, genotype analysis was performed by PCR on isolated genomic DNA (5F and 5R2). F2 heterozygous mice genotyping was done by Transnetyx. Mice used in the study were the offspring of crosses between F1 and/or F2 generations (50% 129/SvJ and 50% C57BL/6J genetic background). Mice were treated in accordance with guidelines approved by the Children's Hospital Animal Care and Use Committee. Analysis of Tmem146 mRNAs from different mouse genotypes First strand cDNAs were prepared from 1 μg total RNA of wt , het or null testes using oligo(dT) primers and reverse transcriptase using a Superscript III first strand kit (Invitrogen). The forward primer spanning exon 7 and 8 (5′-CTGACAAACTGAGTCACCTG-3′) and the reverse primer corresponding to exon 12 (5′-GACTGCACATTCACTGTACAC-3′) amplified 561 and 410 bp from the wt and mutant cDNAs, respectively. Western blotting and immunoprecipitation Spermatozoa from the cauda epididymis were washed and suspended in PBS, counted in a hemocytometer, and lyzed directly in 2× Lithium dodecyl sulfate (LDS) sample buffer with 50 mM dithiothreitol. Lysates corresponding to either 5×10 5 or 1×10 6 spermatozoa were analysed by western blotting. Testes were solubilized in lysis buffer (T-PER, Pierce) supplemented with a PIC. Solubilized proteins cleared by centrifugation (14,000 g ) were immunoprecipitated with anti-CATSPER1, CATSPERβ, CATSPERδ786 or CATSPERγ. Proteins were detected with horseradish peroxidase-conjugated anti-rabbit IgG. Flagellar beat and waveform analysis Spermatozoa from dissected cauda epididymis (swim upward method) were collected in HEPES buffered saline (HS) media containing (in mM): 135 NaCl, 5 KCl, 2 CaCl 2 , 1 MgSO 4 , 20 HEPES, 5 glucose, 10 lactic acid, 1 Na pyruvate, pH 7.4 (with NaOH). Spermatozoa were plated on 35 mm coverslips for 15 min (22 °C); unattached sperm were removed by gentle pipette wash (time 0) and basal beat frequencies recorded. Activated motility was recorded within the first 10 min after adding pre-warmed HTF-capacitating medium (in mM): 102 NaCl, 4.7 KCl, 2 CaCl 2 , 0.2 MgCl 2 , 0.37 KH 2 PO 4 , 2.78 glucose, 18.3 lactic acid, 0.33 Na pyruvate, 25 HCO 3 − and 4 mg ml −1 BSA). To induce hyperactivation, attached sperm cells were incubated in human tubal fluid (HTF) media for 90 min at 37 °C (5% CO 2 ). All subsequent images were recorded at room temperature. The flagellar waveform was analysed by stop-motion digital imaging collected at 60 Hz (XCAP image processing software, EPIX; 2 s movies). Beat frequency of each sperm cell was calculated as one-half of the time elapsed for two complete flagellar beats. The bending angle, α, of the sperm tail was measured using ImageJ software. Electrophysiological recording of mouse spermatozoa Whole-cell recording of corpus epididymal spermatozoa from mice 3–5 months of age was performed blinded [1] , [8] . The standard bath solution, HS, is described above. After break-in, the access resistance was 25–80 MΩ. The standard pipette solution was (mM): 115 Cs-Methanesulfonate (Cs-MeSO 3 ), 5 CsCl, 10 Cs 4 -BAPTA, 10 HEPES and 10 MES, pH 7.2 with H-MeSO 3 . I CatSper was measured as a monovalent current in divalent-free conditions (mM): 150 Na-MeSO 3 , 2 Na 3 HEDTA, 2 EGTA and 20 HEPES, pH 7.4 with NaOH. I KSper was recorded in bath solution containing (mM): 150 K-MeSO 3 , 10 K-HEPES and 10 MES (pH 7.4). All experiments were performed at 22–24 °C. All currents were recorded using an Axopatch 200B amplifier, acquired with Clampex (pClamp9) (Molecular Devices) and analysed with Origin software (Originlab). Signals were low pass filtered at 2 kHz and sampled at 10 kHz. Data are mean±s.e.m. Statistical analysis Paired two-tailed ( Fig. 5c ) and unpaired two-tailed (all other) Student's t -tests yielded P -values as listed. How to cite this article: Chung, J.-J. et al . A novel gene required for male fertility and functional CATSPER channel formation in spermatozoa. Nat. Commun. 2:153 doi: 10.1038/ncomms1153 (2011).